Aurora-A controls pre-replicative complex assembly and DNA replication by stabilizing geminin in mitosis Geminin, an essential factor for DNA replication, directly binds to the licensing factor Cdt1 and inhibits pre-replicative complex formation to prevent re-replication. In G1, geminin levels are controlled by the anaphase-promoting complex/cyclosome (APC/C) ubiquitin ligase complex, which targets geminin for proteasomal degradation to allow pre-replicative complex formation. Conversely, from S to G2, geminin is stabilized due to APC/C ubiquitin ligase complex inhibition, ensuring the inhibition of pre-replicative complex formation. However, mitotic regulation of geminin has hitherto not been described. Here we show that Aurora-A phosphorylates geminin on Thr25 during M phase, and this event induces geminin stabilization by preventing its APC/C ubiquitin ligase complex-mediated degradation during mitosis. In turn, stabilized geminin inhibits SCF Skp2 -mediated degradation of Cdt1 to ensure pre-replicative complex formation in the ensuing S phase. The Aurora-A–geminin–Cdt1 axis therefore represents a critical regulator of proper DNA replication. In eukaryotes, DNA replication is restricted to occur only once per cell cycle. Licensing is mediated by the assembly of the pre-replicative complex (pre-RC) on replication origins. The assembly of the essential pre-RC at these origins can only occur between late mitosis and early G1 when cyclin-dependent kinase (CDK) activity is low and anaphase-promoting complex/cyclosome ubiquitin ligase complex (APC/C) activity is high. The pre-RC is composed of the origin recognition complex (ORC), Cdc6, Cdt1 and the mini-chromosome maintenance (MCM) proteins [1] . During late M and early G1, Cdc6 and Cdt1 are loaded onto replication origins in an ORC-dependent manner and subsequently recruit MCM proteins to the origins. Once the pre-RC are assembled, origins are licensed for replication in the subsequent S phase and are ready to fire. Geminin, a known repressor of re-replication, directly binds to Cdt1 and inhibits its function [2] . Furthermore, geminin controls the basal level of Cdt1 and induces its accumulation during mitosis by inhibiting its ubiquitin-dependent proteolysis [2] . Thereby, the depletion of geminin during mitosis causes the destabilization of Cdt1 and subsequently prevents MCM loading in the subsequent G1 (ref. 3 ). Thus, it is proposed that geminin has both negative and positive roles in pre-RC formation, indicating that protein level of geminin must be appropriately and strictly controlled to ensure proper DNA replication. The protein level of geminin is regulated by the ubiquitin-proteasome system; geminin is degraded at the exit of mitosis by the APC/C complex in Xenopus egg extract [4] , whereas it is a target of the APC/C Cdh1 ubiquitin ligase complex in mammalian cells [5] , [6] . The APC/C activity is dependent on its co-activators, Cdc20 and Cdh1, which associate with APC/C during specific periods in the mammalian cell cycle [7] . APC/C Cdc20 is active early in mitosis, and APC/C Cdh1 has an essential role from late M to the G1/S transition [7] . Cdh1 can only activate APC/C once APC/C Cdc20 has decreased the CDK1 activity by initiating cyclin destruction, when Cdh1 has been dephosphorylated by protein phosphatases in late M (ref. 7 ). DNA replication depends on the APC/C-mediated degradation of geminin, which releases the inhibition of Cdt1 incorporation into pre-RCs and permits the proper assembly of these complex components [2] , [8] . Origin firing can only occur after the APC/C is inactivated and CDKs become active. To strictly inhibit the assembly of pre-RC during S–G2 phase, APC/C is inactivated by several mechanisms: binding to its inhibitor Emi1, CDK-mediated phosphorylation of Cdh1 (which blocks its ability to activate APC/C), and degradation of both Cdh1 (ref. 9 ) and its major UBC, namely UbcH10 (ref. 10 ). In this study, we found that Aurora-A phosphorylates geminin to protect it from APC/C during mitosis. In turn, Aurora-A-mediated stabilization of geminin inhibits SCF Skp2 -mediated degradation of Cdt1 to ensure pre-RC formation in the ensuing S phase. Phosphorylation of geminin prevents its degradation Geminin protein levels oscillate during the cell cycle, that is, accumulating in S and disappearing in early G1 ( Supplementary Fig. S1a ). The half-life of geminin in mitosis (mitotic geminin) was elongated compared with that of either asynchronous or G1-synchronized cells (Supplementary Fig. S1b,c), and treatment with the proteasome inhibitor MG132 resulted in geminin protein accumulation in G1 ( Supplementary Fig. S1d ). Geminin is known to be ubiquitylated via APC/C in G1 phase [4] . Recent analyses at the single-cell level by immunocytochemistry have shown the timing of geminin degradation in mitosis, which takes place following cyclin B degradation, in late anaphase [11] . We confirmed that the depletion of Cdh1 stabilized geminin protein ( Supplementary Fig. S1e ). Emi1 is induced by E2F to inactivate APC/C Cdh1 at the G 1 /S transition [12] . At the onset of mitosis, Emi1 is degraded following the phosphorylation by Plk1 and ubiquitylation by SCF β-TrCP , and this allows the activation of APC/C [13] , [14] . Although geminin is absent during G1 and accumulates during S, G2 and M, consistent with the idea that it is an APC/C substrate, geminin is stable even in mitosis after APC/C is activated. These findings led us to hypothesize that geminin may be stabilized during mitosis by a hitherto unknown pathway. We first noted a band shift of geminin during mitosis by immunoblotting ( Supplementary Fig. S1a ). The band shift was eliminated by λ-phosphatase (λ-PPase) treatment ( Fig. 1a ), suggesting that geminin is phosphorylated during mitosis. Therefore, we assumed that phosphorylation is important for geminin stabilization during mitosis. Geminin is a highly conserved protein and has three conserved putative phosphorylation serine/threonine sites, Thr25, Ser32 and Ser60, surrounding the destruction box (D-box) motif that is recognized by APC/C ( Fig. 1b ). To identify the phosphorylation site and further clarify the implication in geminin protein stability, we generated three phospho-mimicking mutants, geminin T25D , geminin S32D and geminin S60D , in which serine/threonine was replaced with aspartic acid. Cells overexpressing either of these mutants were synchronized in M (noc 0 h) and G1 (noc 4 h). These mutants were highly expressed in M, but only geminin T25D was abundant in G1 ( Fig. 1c ). Interestingly, Thr25 is a component of the D-box in geminin ( Fig. 1b ). We also generated a phospho-defective mutant (T25A) by replacing threonine with alanine. We examined the stability of these mutant molecules after the release from nocodazole (Noc) arrest. Geminin T25A was already unstable during M, whereas geminin T25D remained stable during G1 ( Fig. 2a ). We further confirmed this phenomenon through double thymidine block release ( Supplementary Fig. S2a ). In G1 extracts, in vitro -translated geminin T25A degraded faster than wild-type geminin, whereas geminin T25D was stable ( Fig. 2b ). MG132 treatment increased wild-type geminin and geminin T25A , but not geminin T25D , protein levels ( Supplementary Fig. S2b ). These findings suggest that geminin is phosphorylated on Thr25 during mitosis and is degraded via APC/C Cdh1 in G1 phase after dephosphorylation. To demonstrate this hypothesis, we examined the effect of Thr25 phosphorylation on geminin degradation by APC/C Cdh1 . Cdh1 depletion increased wild-type geminin and geminin T25A , but not geminin T25D , protein levels ( Supplementary Fig. S2c ). As Emi1 depletion is known to give rise to ectopic APC/C Cdh1 activation [5] , we attempted to deplete Emi1, resulting in the reduction of wild-type geminin and geminin T25A , but not geminin T25D , protein levels ( Supplementary Fig. S2d ). Moreover, the in vitro ubiquitylation of geminin T25D via APC/C Cdh1 was not detectable, whereas that of wild-type geminin and geminin T25A was observed ( Fig. 2c ). Interestingly, immunoprecipitation analysis revealed that HA-tagged Cdh1 interacted with wild-type geminin and geminin T25A , but not with geminin T25D ( Fig. 2d ), indicating that the inability of geminin T25D to interact with APC/C Cdh1 may explain its resistance to APC/C Cdh1 -dependent proteolysis. 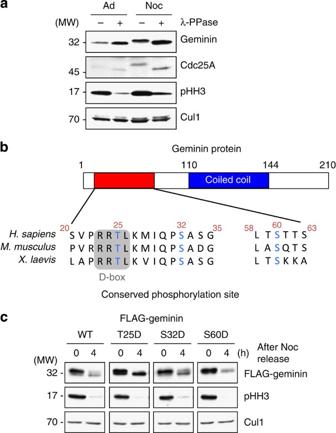Figure 1: Geminin is stabilized during mitosis through the blockade of proteasomal degradation. (a) Noc-arrested HeLa cells were used as arrested mitotic cells (at mitotic shake-off) (Noc) and adherent cells after mitotic shake-off (Ad). Synchronized cell extracts were treated with λ-PPase at 30 °C for 30 min. Cdc25A and phospho-histone H3 (pHH3) were used as controls for phosphorylated proteins. MW, molecular weight in kDa. (b) Candidates for conserved phosphorylation sites in geminin. Geminin phosphorylation sites inHomo sapiens(Thr25, Ser32 and Ser60) are conserved in other species. D-box indicates an APC/CCdh1-recognition site designated as a destruction box. (c) HeLa cells were transfected with either FLAG-tagged wild-type (WT) geminin, gemininT25D, gemininS32Dor gemininS60D. Cells were synchronized by Noc. Cells in M were collected after 0 h from mitotic shake-off. Cells in G1 were collected in G1 after Noc release for 4 h. FLAG-tagged geminin, pHH3 and Cul1 expressions were examined by immunoblotting. MW, molecular weight in kDa. Figure 1: Geminin is stabilized during mitosis through the blockade of proteasomal degradation. ( a ) Noc-arrested HeLa cells were used as arrested mitotic cells (at mitotic shake-off) (Noc) and adherent cells after mitotic shake-off (Ad). Synchronized cell extracts were treated with λ-PPase at 30 °C for 30 min. Cdc25A and phospho-histone H3 (pHH3) were used as controls for phosphorylated proteins. MW, molecular weight in kDa. ( b ) Candidates for conserved phosphorylation sites in geminin. Geminin phosphorylation sites in Homo sapiens (Thr25, Ser32 and Ser60) are conserved in other species. D-box indicates an APC/C Cdh1 -recognition site designated as a destruction box. ( c ) HeLa cells were transfected with either FLAG-tagged wild-type (WT) geminin, geminin T25D , geminin S32D or geminin S60D . Cells were synchronized by Noc. Cells in M were collected after 0 h from mitotic shake-off. Cells in G1 were collected in G1 after Noc release for 4 h. FLAG-tagged geminin, pHH3 and Cul1 expressions were examined by immunoblotting. MW, molecular weight in kDa. 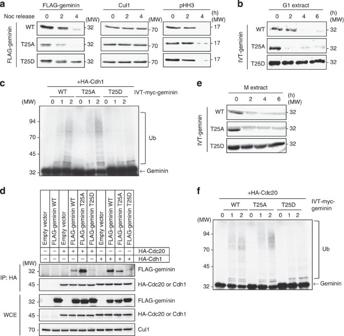Figure 2: Phosphorylation of geminin on Thr25 during mitosis prevents its proteasomal degradation by both APC/CCdh1and APC/CCdc20. (a) HeLa cells were transfected with either wild-type (WT) geminin, gemininT25Aor gemininT25D, and synchronized in M–G1 by Noc. Cells were collected at 0, 2 and 4 h after mitotic shake-off. FLAG-tagged geminin, phospho-histone H3 (pHH3) and Cul1 expressions were examined by immunoblotting. (b) The half-life of IVT-myc-tagged geminin proteins (WT, T25A and T25D) were examined by thein vitrodegradation assay. Cell extracts were obtained from synchronized HeLa cells in G1 (5 h after mitotic shake-off). Cell lysates with IVT-myc-tagged geminin protein were incubated for the indicated times. IVT-myc-tagged geminin protein expression was examined by immunoblotting with an anti-myc antibody. (c) Anin vitroubiquitylation assay was performed using35S-labelled IVT-geminin WT, gemininT25Aor gemininT25D, and immunopurified APC/CCdh1from HeLa cells.35S-labelled IVT-geminin protein was incubated for the indicated times at 30 °C. The abundance of35S-labelled IVT-geminin proteins was detected by autoradiography. (d) FLAG-tagged geminin WT, gemininT25Aor gemininT25D, with or without HA-tagged Cdc20 or Cdh1, were transfected into 293T cells. After 24 h, cells were treated with 25 μM MG132 for 7 h. Cell extracts were immunoprecipitated with an anti-HA antibody, and blotted with an anti-FLAG antibody and an anti-HA antibody. IP, immunoprecipitation; MW, molecular weight in kDa; WCE, whole cell extracts. (e) The half-life of IVT-myc-tagged geminin proteins (WT, T25A and T25D) was examined by thein vitrodegradation assay. Cell extracts were obtained from synchronized HeLa cells in M (at mitotic shake-off). Cell lysates were incubated with IVT-myc-tagged geminin protein for the indicated times. IVT-myc-tagged geminin protein expression was examined by immunoblotting with an anti-myc antibody. (f) Anin vitroubiquitylation assay was performed using35S-labelled IVT-geminin WT, gemininT25Aor gemininT25D, and immunopurified APC/CCdc20from HeLa cells.35S-labelled IVT-geminin proteins were incubated for the indicated times at 30 °C. The abundance of these proteins was detected by autoradiography. MW, molecular weight in kDa. Full size image Figure 2: Phosphorylation of geminin on Thr25 during mitosis prevents its proteasomal degradation by both APC/C Cdh1 and APC/C Cdc20 . ( a ) HeLa cells were transfected with either wild-type (WT) geminin, geminin T25A or geminin T25D , and synchronized in M–G1 by Noc. Cells were collected at 0, 2 and 4 h after mitotic shake-off. FLAG-tagged geminin, phospho-histone H3 (pHH3) and Cul1 expressions were examined by immunoblotting. ( b ) The half-life of IVT-myc-tagged geminin proteins (WT, T25A and T25D) were examined by the in vitro degradation assay. Cell extracts were obtained from synchronized HeLa cells in G1 (5 h after mitotic shake-off). Cell lysates with IVT-myc-tagged geminin protein were incubated for the indicated times. IVT-myc-tagged geminin protein expression was examined by immunoblotting with an anti-myc antibody. ( c ) An in vitro ubiquitylation assay was performed using 35 S-labelled IVT-geminin WT, geminin T25A or geminin T25D , and immunopurified APC/C Cdh1 from HeLa cells. 35 S-labelled IVT-geminin protein was incubated for the indicated times at 30 °C. The abundance of 35 S-labelled IVT-geminin proteins was detected by autoradiography. ( d ) FLAG-tagged geminin WT, geminin T25A or geminin T25D , with or without HA-tagged Cdc20 or Cdh1, were transfected into 293T cells. After 24 h, cells were treated with 25 μM MG132 for 7 h. Cell extracts were immunoprecipitated with an anti-HA antibody, and blotted with an anti-FLAG antibody and an anti-HA antibody. IP, immunoprecipitation; MW, molecular weight in kDa; WCE, whole cell extracts. ( e ) The half-life of IVT-myc-tagged geminin proteins (WT, T25A and T25D) was examined by the in vitro degradation assay. Cell extracts were obtained from synchronized HeLa cells in M (at mitotic shake-off). Cell lysates were incubated with IVT-myc-tagged geminin protein for the indicated times. IVT-myc-tagged geminin protein expression was examined by immunoblotting with an anti-myc antibody. ( f ) An in vitro ubiquitylation assay was performed using 35 S-labelled IVT-geminin WT, geminin T25A or geminin T25D , and immunopurified APC/C Cdc20 from HeLa cells. 35 S-labelled IVT-geminin proteins were incubated for the indicated times at 30 °C. The abundance of these proteins was detected by autoradiography. MW, molecular weight in kDa. Full size image Geminin T25A protein levels were lower than wild-type geminin protein levels at prometaphase ( Fig. 2a ), whereas in vitro -translated wild-type geminin, which was not phosphorylated on Thr25, and geminin T25A were degraded in mitotic extracts ( Fig. 2e ), suggesting that phosphorylated geminin is protected from degradation via APC/C Cdc20 . As expected, the in vitro ubiquitylation of geminin T25D via APC/C Cdc20 was not detectable ( Fig. 2f ). Moreover, HA-Cdc20 interacted with wild-type geminin and geminin T25A , but not with geminin T25D ( Fig. 2d ). Thus, phosphorylation of geminin on Thr25 also protects it from APC/C Cdc20 -mediated proteolysis in mitosis. Next, to elucidate the physiological role of geminin phosphorylation on Thr25, we generated an antibody against geminin phosphorylated on Thr25. The λ-PPase treatment almost completely eliminated the recognition of geminin in mitotic extracts by this antibody ( Supplementary Fig. S3a ). Moreover, this antibody recognized the wild-type geminin, but not geminin T25A ( Supplementary Fig. S3b ). We then used this antibody to probe for geminin phosphorylated on Thr25 at M and G1 phase. Thr25 phosphorylation of endogenous geminin was detectable exclusively in mitosis ( Supplementary Fig. S3c ). Thr25 of geminin is phosphorylated by Aurora-A To further deepen the understanding of geminin phosphorylation, we identified which kinase phosphorylates geminin on Thr25. We found that amino acids 23–26 (RRTL) within the D-box (which include Thr25) matched the consensus sequences (R-X-S/T-L/V) for phosphorylation by Aurora-A, a known mitotic kinase ( Fig. 3a ). The serine/threonine kinase Aurora-A is essential for mitotic entry, centrosome duplication, spindle formation, chromosome segregation and cytokinesis [15] . Geminin was co-localized with Aurora-A through mitotic progression ( Fig. 3b and Supplementary Fig. S4a ), but Aurora-A and phosphorylated geminin disappeared together in the G1 ( Supplementary Fig. S4b ). Interestingly, APC/C Cdh1 targets Aurora-A for the destruction at mitotic exit [16] . 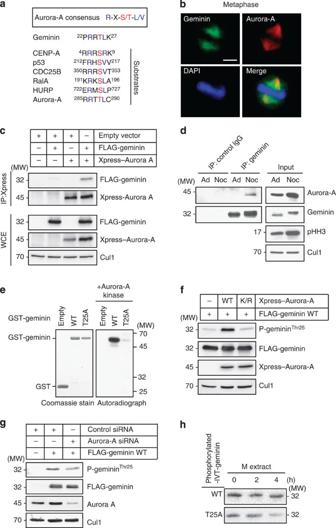Figure 3: Phosphorylation of geminin on Thr25 by Aurora-A kinase during mitosis. (a) Comparison of the amino acid sequences of human geminin from 22 to 27 with those of phosphorylation sites of other known Aurora-A substrates. (b) Subcellular co-localization of geminin and Aurora-A during mitosis. Expression of geminin (green) and Aurora-A (red) was visualized in HeLa cells by immunofluorescence analysis. Scale bar, 5 μm. (c) FLAG-tagged geminin wild-type (WT) or empty vector was transfected into 293T cells with or without Xpress-tagged Aurora-A. Cell lysates were immunoprecipitated with an anti-Xpress antibody. IP, immunoprecipitation; MW, molecular weight in kDa; WCE, whole cell extracts. (d) Noc-arrested HeLa cells were used as arrested mitotic cells (at mitotic shake-off) and adherent cells after mitotic shake-off. Cell lysates were immunoprecipitated with an anti-geminin polyclonal antibody. Noc, arrested mitotic cells (at mitotic shake-off); Ad, adherent cells after mitotic shake-off; pHH, phospho-histone H3 (pHH3). (e)In vitroAurora-A kinase assay using GST-tagged recombinant geminin protein (WT or T25A) and γ32p-ATP. The phosphorylation was detected by autoradiography. (f)In vivoAurora-A kinase assay using 293T cells transfected with Xpress-tagged Aurora-A WT or the kinase-dead mutant (K/R). After 24 h, cells were collected and lysed. Phosphorylation status was examined by immunoblotting with an anti-phosphorylated geminin Thr25-specific antibody (P-gemininThr25). (g) Levels of geminin phosphorylation on Thr25 in Aurora-A-depleted cells. 293T cells were co-transfected with FLAG-tagged geminin WT and control or Aurora-A siRNA. Expression of phospho-geminin (P-gemininThr25), FLAG-tagged geminin, Aurora-A and Cul1 was examined by immunoblotting. (h) The half-life of IVT-myc-tagged geminin proteins (WT and T25A) after Aurora-A-mediated phosphorylation was examined by anin vitrodegradation assay. Cell extracts were obtained from synchronized HeLa cells in M phase (at mitotic shake-off). IVT-myc-tagged geminin protein (WT or T25A) was incubated with recombinant Aurora-A protein in kinase buffer at 30 °C for 1 h. Then, IVT-myc-tagged geminin protein was incubated with cell lysates for the indicated times. Expression of IVT-myc-tagged geminin protein was examined by immunoblotting with an anti-myc antibody. MW, molecular weight in kDa. Figure 3: Phosphorylation of geminin on Thr25 by Aurora-A kinase during mitosis. ( a ) Comparison of the amino acid sequences of human geminin from 22 to 27 with those of phosphorylation sites of other known Aurora-A substrates. ( b ) Subcellular co-localization of geminin and Aurora-A during mitosis. Expression of geminin (green) and Aurora-A (red) was visualized in HeLa cells by immunofluorescence analysis. Scale bar, 5 μm. ( c ) FLAG-tagged geminin wild-type (WT) or empty vector was transfected into 293T cells with or without Xpress-tagged Aurora-A. Cell lysates were immunoprecipitated with an anti-Xpress antibody. IP, immunoprecipitation; MW, molecular weight in kDa; WCE, whole cell extracts. ( d ) Noc-arrested HeLa cells were used as arrested mitotic cells (at mitotic shake-off) and adherent cells after mitotic shake-off. Cell lysates were immunoprecipitated with an anti-geminin polyclonal antibody. Noc, arrested mitotic cells (at mitotic shake-off); Ad, adherent cells after mitotic shake-off; pHH, phospho-histone H3 (pHH3). ( e ) In vitro Aurora-A kinase assay using GST-tagged recombinant geminin protein (WT or T25A) and γ 32p -ATP. The phosphorylation was detected by autoradiography. ( f ) In vivo Aurora-A kinase assay using 293T cells transfected with Xpress-tagged Aurora-A WT or the kinase-dead mutant (K/R). After 24 h, cells were collected and lysed. Phosphorylation status was examined by immunoblotting with an anti-phosphorylated geminin Thr25-specific antibody (P-geminin Thr25 ). ( g ) Levels of geminin phosphorylation on Thr25 in Aurora-A-depleted cells. 293T cells were co-transfected with FLAG-tagged geminin WT and control or Aurora-A siRNA. Expression of phospho-geminin (P-geminin Thr25 ), FLAG-tagged geminin, Aurora-A and Cul1 was examined by immunoblotting. ( h ) The half-life of IVT-myc-tagged geminin proteins (WT and T25A) after Aurora-A-mediated phosphorylation was examined by an in vitro degradation assay. Cell extracts were obtained from synchronized HeLa cells in M phase (at mitotic shake-off). IVT-myc-tagged geminin protein (WT or T25A) was incubated with recombinant Aurora-A protein in kinase buffer at 30 °C for 1 h. Then, IVT-myc-tagged geminin protein was incubated with cell lysates for the indicated times. Expression of IVT-myc-tagged geminin protein was examined by immunoblotting with an anti-myc antibody. MW, molecular weight in kDa. Full size image We then investigated the direct interaction between geminin and Aurora-A. FLAG-tagged geminin co-immunoprecipitated with Xpress-tagged Aurora-A ( Fig. 3c ). Moreover, the endogenous interaction between Aurora-A and geminin was observed in mitosis, but not in interphase ( Fig. 3d ). Thus, Aurora-A exhibited mitosis-specific interaction with geminin. To determine the ability of Aurora-A to phosphorylate geminin, we performed an in vitro kinase assay. Aurora-A strongly phosphorylated purified wild-type glutathione S- transferase (GST)–geminin, but not GST–geminin T25A ( Fig. 3e ). Moreover, a kinase-dead mutant (K162R) of Aurora-A displayed significantly reduced ability to phosphorylate geminin at Thr25, which further highlights the specificity of Aurora-A-mediated geminin phosphorylation ( Fig. 3f ). In fact, geminin phosphorylated on Thr25 co-localized with Aurora-A in mitotic cells ( Supplementary Fig. S4b ). Moreover, the depletion of Aurora-A impaired geminin phosphorylation ( Fig. 3g ). As shown in Fig. 2e , wild-type geminin and geminin T25A were degraded in mitotic extracts, whereas wild-type geminin but not geminin T25A was stabilized in mitotic extracts after in vitro phosphorylation by Aurora-A ( Fig. 3h ). Moreover, a shorter half-life of geminin was observed in Noc-arrested cells after Aurora-A depletion ( Supplementary Fig. S5 ). Cdc20 depletion stabilized geminin in mitotic Aurora-A-depleted cells ( Supplementary Fig. S5 ), indicating that Aurora-A-mediated geminin phosphorylation prevents geminin degradation by APC/C Cdc20 at prometaphase. Phosphorylated geminin stabilizes Cdt1 in mitosis We then investigated the physiological role of geminin phosphorylation during mitosis. A previous report indicated that the inhibition of geminin synthesis during mitosis leads to impaired pre-RC formation and DNA replication in the ensuing cell cycle, and that geminin binds and protects Cdt1 from proteasome-dependent degradation to ensure the accumulation of Cdt1 in G 2 and M (ref. 3 ). Similarly, Cdt1 was reported to be rapidly downregulated after geminin was silenced in Drosophila cells [17] . As shown by previous studies [3] , [18] , we confirmed that Cdt1 was hyperphosphorylated in mitosis and did not bind to chromatin ( Supplementary Fig. S6 ). Moreover, dephosphorylation of Cdt1 coincided with chromatin association ( Supplementary Fig. S6 ). A previous report revealed that the inhibition of CDK1 in mitosis induced an increase in the chromatin-associated Cdt1 fraction to the expense of the soluble Cdt1, and that geminin bound with Cdt1 interfered with this binding to the chromatin [3] . These findings suggest that Cdt1 recruitment to chromatin may be regulated by dephosphorylation in late M. Interestingly, geminin downregulation and Cdt1 recruitment to chromatin occur simultaneously ( Supplementary Fig. S6 ). To understand the role of geminin in Cdt1 recruitment to chromatin, we examined whether mitotic depletion of geminin affected Cdt1 recruitment to chromatin ( Fig. 4a ). Consistent with that published before [3] , mitotic depletion of geminin decreased the levels of both soluble and chromatin-associated Cdt1 and impaired MCM6 loading ( Fig. 4b ). Interestingly, mitotic depletion of Aurora-A induced a similar decrease in the level of both soluble and chromatin-associated Cdt1 ( Fig. 4c ). These findings suggest that geminin phosphorylated by Aurora-A stabilizes soluble Cdt1, which, in turn, is recruited to the chromatin. In contrast to what was observed when geminin was depleted during interphase [19] , mitotic depletion of geminin or Aurora-A did not induce the DNA damage response, as shown by the lack of Chk2 phosphorylation ( Supplementary Fig. S7 ). Moreover, the protein level and kinase activity of Aurora-A were not affected by the depletion of mitotic geminin (data not shown), and the phosphorylation of geminin on Thr25 did not affect its interaction with Cdt1 ( Supplementary Fig. S8a ). 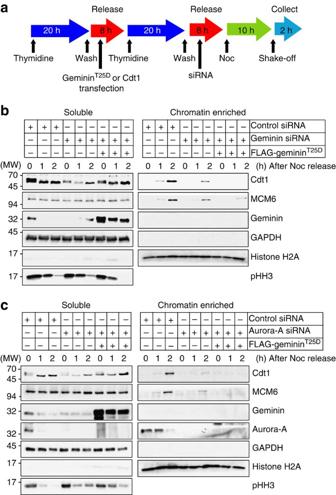Figure 4: Geminin stabilization during mitosis controls pre-RC formation. (a) Experimental outline for the synchronization of U2OS cells. Cells were synchronized with double thymidine block as indicated schedule. G1/S-arrested cells were released and transfected with siRNA for 8 h, followed by Noc treatment for 12 h. Mitotic cells were collected by shake-off and released for indicated time. (b) Geminin depletion during mitosis impaired licensing at mitotic exit. U2OS cells were treated with geminin siRNA during release from the second thymidine block and collected at 0, 1 and 2 h after release from the Noc block as described ina. After release from the first thymidine block, cells were transfected with FLAG-tagged gemininT25D. The soluble and chromatin fractions were separated and immunoblotted for the indicated proteins. MW, molecular weight in kDa; GAPDH, glyceraldehyde 3-phosphate dehydrogenase; pHH, phospho-histone H3 (pHH3). (c) Aurora-A depletion during mitosis impaired licensing at mitotic exit. U2OS cells were treated with Aurora-A siRNA during release from the second thymidine block and collected at 0, 1 and 2 h after release from the Noc block as described ina. After release from the first thymidine block, cells were transfected with FLAG-tagged gemininT25D. The soluble and chromatin fractions were separated and immunoblotted for the indicated proteins. MW, molecular weight in kDa. Figure 4: Geminin stabilization during mitosis controls pre-RC formation. ( a ) Experimental outline for the synchronization of U2OS cells. Cells were synchronized with double thymidine block as indicated schedule. G1/S-arrested cells were released and transfected with siRNA for 8 h, followed by Noc treatment for 12 h. Mitotic cells were collected by shake-off and released for indicated time. ( b ) Geminin depletion during mitosis impaired licensing at mitotic exit. U2OS cells were treated with geminin siRNA during release from the second thymidine block and collected at 0, 1 and 2 h after release from the Noc block as described in a . After release from the first thymidine block, cells were transfected with FLAG-tagged geminin T25D . The soluble and chromatin fractions were separated and immunoblotted for the indicated proteins. MW, molecular weight in kDa; GAPDH, glyceraldehyde 3-phosphate dehydrogenase; pHH, phospho-histone H3 (pHH3). ( c ) Aurora-A depletion during mitosis impaired licensing at mitotic exit. U2OS cells were treated with Aurora-A siRNA during release from the second thymidine block and collected at 0, 1 and 2 h after release from the Noc block as described in a . After release from the first thymidine block, cells were transfected with FLAG-tagged geminin T25D . The soluble and chromatin fractions were separated and immunoblotted for the indicated proteins. MW, molecular weight in kDa. Full size image Next, we examined whether introducing ectopic geminin T25D rescued the downregulation of soluble Cdt1 protein at M phase in geminin- or Aurora-A-depleted cells. As we used siRNA targeting the 3′-untranslated region region to deplete geminin, exogenous geminin expression was not affected by this siRNA ( Supplementary Fig. S8b ). Interestingly, ectopic geminin T25D in geminin- or Aurora-A-depleted cells induced a stabilization of soluble Cdt1 in M ( Fig. 4b ). As expected, the loading of Cdt1 and MCM in G1 was suppressed by ectopic geminin T25D ( Fig. 4b ), indicating that phosphorylated geminin, which cannot be degraded via APC/C, prevents Cdt1 from loading onto chromatin during M. Indeed, ectopic Cdt1 rescued the impairment of MCM loading in geminin- or Aurora-A-depleted cells ( Fig. 5a ). Moreover, the depletion of geminin or Aurora-A in mitosis suppressed 5-bromodeoxyuridine (BrdU) incorporation in the ensuing S phase ( Supplementary Fig. S9a,b and Fig. 5c ), even though the kinetics of mitotic exit was not affected, as shown by the phosphorylation of histone H3 on Ser10 ( Figs 4b , c and ) and fluorescence-activated cell sorting analysis ( Supplementary Figs S10 and S11 ). Ectopic geminin T25D in geminin- or Aurora-A-depleted cells could not rescue BrdU incorporation in the ensuing S phase ( Supplementary Fig. S9a,b ). This is likely due to the impairment of Cdt1 and MCM6 loading ( Fig. 4b ). Interestingly, ectopic Cdt1 in geminin- or Aurora-A-depleted cells rescued BrdU incorporation in the ensuing S phase ( Fig. 5c ). These findings suggest that strict regulation of geminin and Cdt1 protein levels depending on the cell cycle phase may be essential for DNA replication. 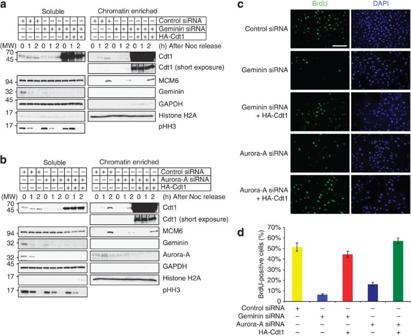Figure 5: Depletion of geminin or Aurora-A during mitosis impaired DNA replication. (a) Geminin depletion during mitosis impaired licensing at mitotic exit. U2OS cells were treated with geminin siRNA during release from the second thymidine block and collected at 0, 1 and 2 h after release from the Noc block as described inFig. 4a. After release from the first thymidine block, cells were transfected with HA-tagged Cdt1. The soluble and chromatin fractions were separated and immunoblotted for the indicated proteins. MW, molecular weight in kDa; GAPDH, glyceraldehyde 3-phosphate dehydrogenase; pHH, phospho-histone H3 (pHH3). (b) Aurora-A depletion during mitosis impaired licensing at mitotic exit. U2OS cells were treated with Aurora-A siRNA during release from the second thymidine block and collected at 0, 1 and 2 h after release from the Noc block as described inFig. 4a. After release from the first thymidine block, cells were transfected with HA-tagged Cdt1. The soluble and chromatin fractions were separated and immunoblotted for the indicated proteins. MW, molecular weight in kDa. (c) U2OS cells plated on glass coverslips were synchronized as described inFig. 4aand labelled with BrdU for 30 min at 10.5 h after release from the Noc block. Cells were then fixed and stained for BrdU (green) by indirect immunofluorescence analysis. Figure shows representative images obtained by indirect immunofluorescence analysis of the cells. The cell nuclei were stained with DAPI (4′,6-diamidino-2-phenylindole; blue). Scale bar, 200 μm. (d) Graph shows the average number of BrdU-positive cells in geminin or Aurora-A mitotic-depleted cells with or without HA-tagged Cdt1. Three independent counts (n=150 cells each count) were used to calculate mean±s.d. Figure 5: Depletion of geminin or Aurora-A during mitosis impaired DNA replication. ( a ) Geminin depletion during mitosis impaired licensing at mitotic exit. U2OS cells were treated with geminin siRNA during release from the second thymidine block and collected at 0, 1 and 2 h after release from the Noc block as described in Fig. 4a . After release from the first thymidine block, cells were transfected with HA-tagged Cdt1. The soluble and chromatin fractions were separated and immunoblotted for the indicated proteins. MW, molecular weight in kDa; GAPDH, glyceraldehyde 3-phosphate dehydrogenase; pHH, phospho-histone H3 (pHH3). ( b ) Aurora-A depletion during mitosis impaired licensing at mitotic exit. U2OS cells were treated with Aurora-A siRNA during release from the second thymidine block and collected at 0, 1 and 2 h after release from the Noc block as described in Fig. 4a . After release from the first thymidine block, cells were transfected with HA-tagged Cdt1. The soluble and chromatin fractions were separated and immunoblotted for the indicated proteins. MW, molecular weight in kDa. ( c ) U2OS cells plated on glass coverslips were synchronized as described in Fig. 4a and labelled with BrdU for 30 min at 10.5 h after release from the Noc block. Cells were then fixed and stained for BrdU (green) by indirect immunofluorescence analysis. Figure shows representative images obtained by indirect immunofluorescence analysis of the cells. The cell nuclei were stained with DAPI (4′,6-diamidino-2-phenylindole; blue). Scale bar, 200 μm. ( d ) Graph shows the average number of BrdU-positive cells in geminin or Aurora-A mitotic-depleted cells with or without HA-tagged Cdt1. Three independent counts ( n =150 cells each count) were used to calculate mean±s.d. Full size image Phosphorylated geminin interferes with Cdt1 degradation We investigated why soluble Cdt1 protein becomes unstable when geminin is depleted in mitosis. Treatment with MG132 or the neddylation inhibitor MLN4924 increased the soluble Cdt1 levels in mitotic geminin- or Aurora-A-depleted cells ( Fig. 6a ), suggesting that soluble Cdt1 downregulation in response to the mitotic depletion of geminin or Aurora-A may be caused by ubiquitin-dependent proteolysis. During S and G2, human Cdt1 is recognized for proteolysis by two distinct E3 ubiquitin ligases, SCF Skp2 and CRL4 Cdt2 (ref. 20 ). It has been demonstrated that Cdt1 is degraded via CRL4 Cdt2 in geminin-depleted cells because of the DNA damage response [21] . We also found that geminin depletion induced Thr68 phosphorylation of Chk2, which is phosphorylated by ataxia telangiectasia mutated (ATM)/ATM and Rad3-related (ATR) after DNA damage ( Supplementary Fig. S7 ). However, geminin depletion in mitosis did not induce DNA damage ( Supplementary Fig. S7 ). These findings suggest that Cdt1 may not be ubiquitylated by CRL4 Cdt2 in mitotic geminin-depleted cells. Indeed, Skp2 depletion, but not Cdt2 depletion, remarkably increased the soluble Cdt1 protein levels ( Fig. 6c ). Accordingly, Skp2 depletion rescued the levels of both soluble and chromatin-associated Cdt1 due to the mitotic depletion of geminin or Aurora-A ( Fig. 7a and b ). In mitotic geminin-depleted cells, Cdt1 expression was increased by the introduction of ectopic FLAG-geminin in an amount-dependent manner ( Fig. 7c ). SCF Skp2 -dependent in vitro ubiquitylation of Cdt1 was inhibited by adding in vitro -translated geminin protein ( Fig. 7d ). Cdt1 T29A , in the presence of which CDK phosphorylation and Skp2 binding are impaired [22] , was not ubiquitylated by SCF Skp2 ( Fig. 7d ). These findings indicate that in mitosis, geminin may protect soluble Cdt1 from SCF Skp2 -dependent degradation for pre-RC formation. 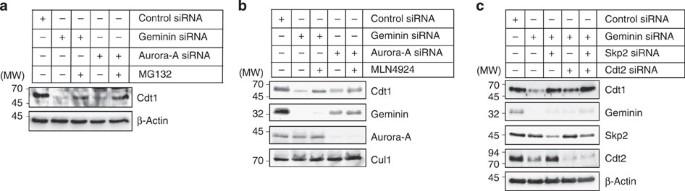Figure 6: Downregulation of Cdt1 by geminin or Aurora-A mitotic depletion is caused by SCFSkp2. (a) U2OS cells were treated with geminin or Aurora-A siRNA during release from the second thymidine block and collected immediately after release from the Noc block as described inFig. 4a. Cells were treated with 25 μM MG132 for 5 h before mitotic shake-off. The soluble fraction was separated and immunoblotted for the indicated proteins. MW, molecular weight in kDa. (b) U2OS cells were treated with geminin or Aurora-A siRNA during release from the second thymidine block and collected immediately after release from the Noc block as described inFig. 4a. Cells were treated with 1 μM MLN4924 for 2 h before mitotic shake-off. The soluble fraction was separated and immunoblotted for the indicated proteins. (c) U2OS cells were treated with geminin siRNA, with or without Skp2 or Cdt2 siRNA, during release from the second thymidine block and collected immediately after release from the Noc block as described inFig. 4a. The soluble fraction was separated and immunoblotted for the indicated proteins. MW, molecular weight in kDa. Figure 6: Downregulation of Cdt1 by geminin or Aurora-A mitotic depletion is caused by SCF Skp2 . ( a ) U2OS cells were treated with geminin or Aurora-A siRNA during release from the second thymidine block and collected immediately after release from the Noc block as described in Fig. 4a . Cells were treated with 25 μM MG132 for 5 h before mitotic shake-off. The soluble fraction was separated and immunoblotted for the indicated proteins. MW, molecular weight in kDa. ( b ) U2OS cells were treated with geminin or Aurora-A siRNA during release from the second thymidine block and collected immediately after release from the Noc block as described in Fig. 4a . Cells were treated with 1 μM MLN4924 for 2 h before mitotic shake-off. The soluble fraction was separated and immunoblotted for the indicated proteins. ( c ) U2OS cells were treated with geminin siRNA, with or without Skp2 or Cdt2 siRNA, during release from the second thymidine block and collected immediately after release from the Noc block as described in Fig. 4a . The soluble fraction was separated and immunoblotted for the indicated proteins. MW, molecular weight in kDa. 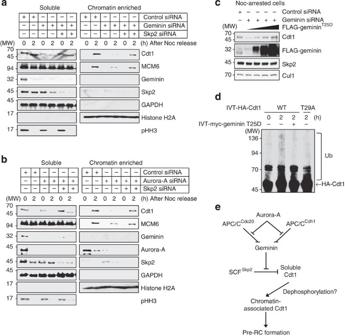Figure 7: Geminin or Aurora-A depletion during mitosis induces SCFSkp2-dependent proteolysis of soluble Cdt1 protein. (a) Geminin depletion during mitosis impaired licensing at mitotic exit. U2OS cells were treated with geminin and/or Skp2 siRNA during release from the second thymidine block and collected at 0 and 2 h after release from the Noc block as described inFig. 4a. The soluble and chromatin fractions were separated and immunoblotted for the indicated proteins. MW, molecular weight in kDa; GAPDH, glyceraldehyde 3-phosphate dehydrogenase; pHH, phospho-histone H3 (pHH3). (b) Aurora-A depletion during mitosis impaired licensing at mitotic exit. U2OS cells were treated with Aurora-A and/or Skp2 siRNA during release from the second thymidine block and collected at 0 and 2 h after release from the Noc block. Soluble and chromatin fractions were separated and immunoblotted for the indicated proteins. (c) Cells were treated with the geminin siRNA during release from second thymidine block and collected immediately after mitotic shake-off. After release from the first thymidine block, cells were transfected with 0.5, 1 or 2 μg of FLAG-tagged gemininT25D. Cdt1, FLAG-tagged geminin, Skp2 and Cul1 expression was examined by immunoblotting. (d) Anin vitroubiquitylation assay was performed using wild-type (WT) or T29A mutant IVT-HA-tagged Cdt1 and immunopurified SCFSkp2from 293T cells. WT IVT-HA-tagged Cdt1 protein was incubated with or without IVT-myc-tagged gemininT25Dprotein for the indicated times. As a negative control, IVT-HA-tagged Cdt1T29Aprotein known as a non-degradable mutant for SCFSkp2-mediated degradation was also used. The abundance of IVT-HA-tagged Cdt1 was detected by SDS–PAGE with a HA antibody. (e) Schematic model for pre-RC formation regulated by the Aurora-A–geminin–Cdt1 axis. Aurora-A protects geminin from APC/CCdc20- and APC/CCdh1-mediated proteolysis through phosphorylation. Phosphorylated geminin may stabilize soluble Cdt1 protein by inhibiting SCFSkp2-mediated proteolysis. Stabilized soluble Cdt1 may load onto chromatin after dephosphorylation and then form the pre-RC. MW, molecular weight in kDa. Full size image Figure 7: Geminin or Aurora-A depletion during mitosis induces SCF Skp2 -dependent proteolysis of soluble Cdt1 protein. ( a ) Geminin depletion during mitosis impaired licensing at mitotic exit. U2OS cells were treated with geminin and/or Skp2 siRNA during release from the second thymidine block and collected at 0 and 2 h after release from the Noc block as described in Fig. 4a . The soluble and chromatin fractions were separated and immunoblotted for the indicated proteins. MW, molecular weight in kDa; GAPDH, glyceraldehyde 3-phosphate dehydrogenase; pHH, phospho-histone H3 (pHH3). ( b ) Aurora-A depletion during mitosis impaired licensing at mitotic exit. U2OS cells were treated with Aurora-A and/or Skp2 siRNA during release from the second thymidine block and collected at 0 and 2 h after release from the Noc block. Soluble and chromatin fractions were separated and immunoblotted for the indicated proteins. ( c ) Cells were treated with the geminin siRNA during release from second thymidine block and collected immediately after mitotic shake-off. After release from the first thymidine block, cells were transfected with 0.5, 1 or 2 μg of FLAG-tagged geminin T25D . Cdt1, FLAG-tagged geminin, Skp2 and Cul1 expression was examined by immunoblotting. ( d ) An in vitro ubiquitylation assay was performed using wild-type (WT) or T29A mutant IVT-HA-tagged Cdt1 and immunopurified SCF Skp2 from 293T cells. WT IVT-HA-tagged Cdt1 protein was incubated with or without IVT-myc-tagged geminin T25D protein for the indicated times. As a negative control, IVT-HA-tagged Cdt1 T29A protein known as a non-degradable mutant for SCF Skp2 -mediated degradation was also used. The abundance of IVT-HA-tagged Cdt1 was detected by SDS–PAGE with a HA antibody. ( e ) Schematic model for pre-RC formation regulated by the Aurora-A–geminin–Cdt1 axis. Aurora-A protects geminin from APC/C Cdc20 - and APC/C Cdh1 -mediated proteolysis through phosphorylation. Phosphorylated geminin may stabilize soluble Cdt1 protein by inhibiting SCF Skp2 -mediated proteolysis. Stabilized soluble Cdt1 may load onto chromatin after dephosphorylation and then form the pre-RC. MW, molecular weight in kDa. Full size image In this study, we describe a novel regulation of geminin during mitosis ( Fig. 7e and Supplementary Fig. S12 ). Aurora-A phosphorylates geminin on Thr25 for it from protecting APC/C-dependent proteolysis. Importantly, stabilized mitotic geminin ensures pre-RC formation by protecting Cdt1 from SCF Skp2 -dependent proteolysis. The pre-RC formation regulated by the Aurora-A–geminin–Cdt1 axis leads to proper DNA replication. The APC/C complex distinctively targets specific substrates and it is tightly regulated to adjust the critical timing of substrate destruction [7] . However, it is still unclear how activated APC/C specifically degrades each of a large number of substrates. In fact, all its substrates are not necessarily degraded simultaneously by APC/C, even though APC/C becomes active during mitosis. The timing of the ubiquitylation of the substrates is tightly regulated by the following mechanisms: (i) protein modification, such as phosphorylation or acetylation, protects the substrates from APC/C [16] , [23] , [24] , [25] , [26] ; (ii) intrinsic regulation of APC/C by substrate ordering influences kinetic differences in the process of ubiquitylation [27] ; and (iii) the binding of proteins with APC/C substrates inhibits ubiquitylation [28] . Phosphorylation protects Cdc6, Aurora-A, Skp2 and geminin from APC/C-mediated degradation [16] , [23] , [24] , [25] . In particular, the inability of phosphorylated Cdc6, Skp2 or geminin to interact with APC/C explains its resistance to APC/C-mediated proteolysis [23] , [25] . Recently, we demonstrated that the phosphorylation of human Aurora-A on Ser51 inhibits its APC Cdh1 -mediated ubiquitylation, and that constitutive phosphorylation on Ser51 is observed in cancer cells with protein overexpression and stabilization [16] . As geminin is highly expressed in certain human cancers [29] , [30] , it will be interesting to examine the involvement of geminin phosphorylation on Thr25 in cancer. Geminin restricts nuclear DNA replication to one round per cell cycle, which ensures genome stability and prevents cells from becoming aneuploid [1] . Re-replication may occur when the pathways controlling pre-RC formation are impaired. Indeed, geminin depletion in mammalian cells is sufficient to cause re-replication [19] , [31] , indicating that geminin has a critical role in replication control. The pre-RC assembly reaction, known as licensing, involves the loading of the Mcm2-7 complex in an ATP-dependent reaction that requires ORC and two essential factors, Cdc6 and Cdt1 (ref. 1 ). It is suggested that the binding of geminin to Cdt1 protects the latter from ubiquitylation and subsequent proteolysis [3] . In this study, we found that introduction of in vitro- translated geminin T25D protein suppressed SCF Skp2 -dependent Cdt1 ubiquitylation ( Fig. 7d ), suggesting that geminin protects soluble Cdt1 from SCF Skp2 -dependent proteolysis by interfering with the binding between Cdt1 and Skp2. However, as Cdt2 depletion slightly increased soluble Cdt1 protein levels ( Fig. 6c ), the possibility of Cdt1 degradation by CRL4 Cdt2 in mitotic geminin-depleted cells cannot be denied. Further detailed studies on the mechanism of inhibition of Cdt1 ubiquitylation may be required. In Xenopus eggs, geminin is suggested to inhibit licensing from S phase to metaphase and seems to be inactivated in interphase through activation of the licensing process [8] , [32] , [33] , [34] . However, a significant proportion of molecules seems to escape degradation at the metaphase–anaphase transition in Xenopus egg extracts [35] , and the Cdt1-inhibiting activity of these remaining molecules must be suppressed through mechanisms other than by proteolysis. Indeed, exogenous geminin associates with and inhibits Cdt1 in the interphase egg extracts [4] , [8] , [35] . Although geminin rapidly disappears at the exit of mitosis and accumulates during S phase in cultured cells [2] , [4] , the remaining pool of geminin in the egg extracts may be regulated by Aurora-A-mediated phosphorylation through escape from APC/C-mediated degradation. It is interesting to examine the precise molecular mechanism of this phenomenon in Xenopus eggs. In S phase, chromatin-associated geminin presents even in the absence of Cdt1, possibly as a precaution to prevent Cdt1 from gaining access to chromatin if it accidentally accumulates during S phase [36] . In this situation, geminin is phosphorylated at Ser45 and Ser49 in HeLa cells [37] , although the physiological relevance of this modification remains to be clarified. Indeed, we identified geminin phosphorylation on Thr25 by Aurora-A kinase during mitosis. In Fig. 1c , the band of geminin T25D was still shifted at G1 similar to that of wild-type geminin and other geminin mutants (geminin S32D and geminin S60D ), suggesting that geminin is phosphorylated at multiple sites during mitosis. These findings indicate that phosphorylation may be important for the functional regulation of geminin in mammalian cells. Furthermore, we found that abundant soluble geminin and Cdt1 protein expression was observed at prometaphase, and that abundant chromatin-associated Cdt1 expression was observed during the G1 phase. Although it is still unclear how the molecular interaction between Cdt1 and geminin can be regulated during M to G1 in mammalian cells, recent studies revealed that (i) the geminin–Cdt1 complex can exist in two distinct forms, a licensing-permissive heterotrimer and a licensing-inhibitory heterohexamer, to regulate a molecular switch between licensing-competent and licensing-defective states in Xenopus and mammalian cells [38] and (ii) the two forms of the Cdt1–geminin complex act as active or inactive complexes for licensing in Xenopus egg extracts [39] . In addition, geminin-mediated nuclear Cdt1 foci formation supports the presence of local interactions between geminin–Cdt1 complexes on chromatin in Xenopus egg extracts [40] . Ode et al. [40] suggested that the higher-order interactions of Cdt1–geminin complexes are cooperatively stabilized on chromatin. Overall, these findings suggest that licensing for proper DNA replication may be strictly regulated by the geminin protein level during cell cycle progression. The amount of geminin, which is determined by Emi1- and Aurora-A-mediated protection from APC/C-mediated proteolysis, may thus be essential for proper DNA replication. Reagents and antibodies Reagents were from the following suppliers: MG132 (Z-Leu-Leu-Leu-CHO) (Peptide Institute Inc., Osaka, Japan); CHX (Sigma); λ-PPase (New England Bio Labs); MLN4924 (Millennium Pharmaceuticals). The geminin phospho-Thr25-specific antibody was generated by immunizing rabbits with the synthetic peptide CVPRR*TLKMIQ, corresponding to amino acids 21–30 of the human geminin sequence, with a phospho-threonine at position 25 (*T). The antibody was purified from serum by two rounds of affinity chromatography, on a phospho-Thr25 peptide column and on a non-phosphopeptide column. The anti-geminin polyclonal antibody was generated using GST fusion recombinant molecules [41] , and the anti-Cdt1 monoclonal antibody was a gift from Dr Kristian Helin (University of Copenhagen). Commercial antibodies were from the following suppliers: anti-p27, anti-Aurora-A and anti-Aurora-B antibodies (Transduction Laboratories); anti-HA (Y-11), anti-cyclin A, anti-cyclin B, anti-MCM6, anti-Cdc25A, anti-Cdc6 and anti-GAPDH antibodies (Santa-Cruz Biotechnology); anti-phospho-Histone H3 (Ser10) antibody (Upstate); anti-Cul1, anti-Emi1, anti-Skp2 and anti-PLK1 antibodies (Zymed); anti-Xpress antibody (Invitrogen); anti-Cdh1 antibody (MBL); anti-geminin (2H7) antibody (Abnova); anti-histone H2A antibody (Abcam); anti-FLAG (M2) and anti-β-actin antibodies (Sigma); anti-phospho-tyrosine antibody (Merck Millipore); anti-Cdt1 and anti-Cdt2 antibodies (Bethyl). Plasmids pEF-FLAG-tagged geminin and pcDNA-HA-tagged Cdt1 were kind gifts from Dr Anindya Dutta (University of Virginia). To produce GST-tagged recombinant proteins, geminin complementary DNA was subcloned into pGEX 4T-1 vectors (GE Healthcare). For in vitro translation, geminin cDNA was also subcloned into pcDNA3.1 His/myc-tagged vectors (Invitrogen). The pcDNA3.1 His/Xpress-tagged Aurora-A was previously described [16] . pCMV HA-tagged Cdt1 and HA-tagged Cdh1 expression vectors were gifts from Dr Kristian Helin (University of Copenhagen). The pEF, pGEX and pcDNA3.1 vectors encoding the FLAG-tagged geminin substitution mutants (T25A and T25D), the pcDNA3.1 vector encoding His/Xpress-tagged Aurora-A kinase-dead mutant (K162R) and the pcDNA3 vector encoding HA-tagged Cdt1 substitution mutant (T29A) were generated using a KOD plus mutagenesis kit (Toyobo). Cell culture and transient transfection HeLa, U2OS and 293T cells were routinely maintained in DMEM (Nissui Pharmaceutical Co. Ltd, Tokyo, Japan) supplemented with 10% heat-inactivated fetal bovine serum (Gibco) and 100 U ml −1 penicillin–streptomycin (Gibco) at 37 °C and 5% CO 2 in air. For experiments, cells were grown to subconfluence in this medium. Transient transfections were performed using FuGENE HD (Roche) following the manufacturer’s instructions. For synchronization, Noc (Sigma) and thymidine (Sigma) were used. HeLa cells were synchronized at prometaphase using 50 ng ml −1 Noc treatment followed by mitotic shake-off. Subsequently, synchronized cells were released from the mitotic arrest by washing out Noc. Adherent cells remaining after mitotic shake-off were also used. Adherent cells dominantly included the cells arrested at G 2 , as confirmed by FACS analysis (data not shown). U2OS were synchronized at the G1/S border by a double thymidine block. In brief, cells were incubated for 20 h in 2 mM thymidine (Sigma), released for 8 h and then incubated for another 20 h in 2 mM thymidine. Immunoprecipitation and immunoblot analysis Cells were transfected with vectors by using FuGENE HD (Roche). Cell lysis and immunoprecipitation were performed as described [13] . Twenty micrograms of protein were subjected to 10% PAGE followed by electroblotting onto a nitrocellulose membrane. To detect the immunocomplex, an ECL Western blotting detection system (Amersham) was used. The immunoprecipitates were subjected to immunoblot analysis. To detect phospho-Thr25 geminin, we performed immunoprecipitation with a phospho-specific antibody against Thr25 of geminin, followed by immunoblotting analysis with a monoclonal antibody against endogenous geminin or an anti-FLAG antibody against FLAG-tagged exogenous geminin. In vitro ubiquitylation assay Ubiquitylation assays were performed as previously described [16] . [ 35 S]methionine-labelled human geminin protein was prepared by coupled transcription–translation reactions in wheat germ extract (Promega). GST-tagged Cdh1 (Abnova) or cold in vitro -translated human Cdc20 protein was also used. The extracts from HeLa cells were immunoprecipitated with an anti-Cdc27 antibody (Sigma). Immunoprecipitants were incubated with Cdh1 or Cdc20 for 1 h at 37 °C and washed four times in QA buffer (10 mM Tris–HCl pH 7.5, 100 mM KCl, 1 mM MgCl 2 , 0.1 mM CaCl 2 , 1 mM dithiothreitol (DTT)). The purified APC/C Cdh1 or APC/C Cdc20 complexes were incubated in reaction mixtures containing the following components in a volume of 7 μl: 40 mM Tris–HCl (pH 7.6), 1 mg ml −1 carboxymethyl BSA, 1 mM DTT, 5 mM MgCl 2 , 10 mM phosphocreatine, 50 μg ml −1 creatine phosphokinase, 0.5 mM ATP, 50 μM ubiquitin, 1 μM ubiquitin aldehyde, 1 pmol of E1, 5 pmol of E2-C, 1 μM okadaic acid and 1–2 pmol of [ 35 S]methionine-labelled human geminin protein. Following incubation at 30 °C for 2 h, samples were loaded for electrophoresis on an 8% polyacrylamide–SDS gel. In vitro ubiquitylation assays for Cdt1 were performed in a volume of 30 μl containing 0.1 μM E1 (Boston Biochem), 10 ng ml −1 Ubch3, 10 ng ml −1 Ubch5c, 1 μM ubiquitin aldehyde, 2.5 μg ml −1 ubiquitin (Sigma) and SCF Skp2 complex in a ubiquitylation buffer (50 mM Tris (pH 7.6), 2 mM ATP, 5 mM MgCl 2 , 0.6 mM DTT, 0.1 μM okadaic acid). In vitro -translated HA-tagged wild-type Cdt1 or Cdt1 T29A was used as the substrate. The reactions were incubated at 30 °C for the indicated times and analysed by SDS–PAGE with an anti-HA antibody. The SCF Skp2 complex was obtained from the lysates of 293T cells after transfection with FLAG-tagged Skp2 together with other SCF components. After 24 h of transfection, cells were incubated with MG132 for 3 h before lysis. Anti-FLAG antibody was used to immunoprecipitate the SCF Skp2 complex. The immunoprecipitants were washed four times in lysis buffer and two times in ubiquitylation reaction buffer (10 mM Tris–HCl pH 7.5, 100 mM NaCl, 5 mM MgCl 2 and 1 mM DTT). Finally, beads were then used for in vitro ubiquitylation assays. Chromatin fractionation For chromatin fractionation, we separated the soluble and insoluble fractions as previously described [42] . Briefly, cells were lysed in CSK buffer and centrifuged for 4 min at 3,200 r.p.m. After centrifugation, the supernatant contained the soluble fraction. The pellet was resuspended in 2 × Laemmli buffer after washing with CSK buffer and then sonicated. This lysate contained the chromatin-enriched fraction. RNA interference The following siRNA oligonucleotides were obtained from Qiagen: geminin, 5′-CCUAUUGCAUUAAAGUACA-3′; Aurora-A, 5′-CACCUUCGGCAUCCUAAUA-3′; and Cdh1, 5′-UCUGGUGGACUGGUCGUCC-3′. Emi1 siRNA was obtained from Dhamacon as the following sequence: 5′-GAUUGUGAUCUCUUAUUAA-3′. Cdt2 siRNA was obtained from Bonac (Kurume, Japan) as the following sequence: 5′-CAAUGGACACCAGAACUCUACCUUU-3′. The negative control (siTrio-negative control siRNA) was obtained from Cosmo Bio Inc. (Tokyo, Japan). Transfections were performed using 20 nM siRNA and Oligofectamine RNAi MAX (Invitrogen), according to the manufacturer’s instructions. In vitro degradation assay For M or G1 extracts, HeLa cells were synchronized in prometaphase by Noc treatment and collected at 0 or 5 h after mitotic shake-off. The collected cells were lysed in hypotonic buffer (25 mM HEPES pH 7.5, 1.5 mM MgCl 2 , 5 mM KCl, 1 mM DTT, 15 mM creatine phosphate, 2 mM ATP) by ten freeze-and-thaw cycles and centrifuged for 5 min at 5,000 r.p.m. and subsequently for 60 min at 13,200 r.p.m. As a substrate, cold IVT-myc-geminin (wild-type, T25A and T25D) was prepared by coupled transcription–translation reactions in wheat germ extracts (Promega). The substrate was incubated in 20 μl of cell extract and a degradation cocktail containing the following components in a volume of 20 μl: 1.5 mg ml −1 ubiquitin, 7.5 mM creatine phosphate, 1 mM ATP, 1 mM MgCl 2 and 25 μg ml −1 CHX. Following incubation at 30 °C for 2, 4 and 6 h, samples were loaded for electrophoresis on a 12% polyacrylamide–SDS gel. Immunofluorescence Cells were grown on glass coverslips, fixed in 4% paraformaldehyde for 10 min and permeabilized with PBS containing 0.1% Triton X-100 for 20 min. After three rinses with PBS, the coverslips were incubated with the primary antibodies. Anti-geminin, anti-geminin phospho-Thr25 and anti-Aurora-A antibodies were used. Alexa Fluor 488-conjugated anti-mouse or rabbit IgG and Alexa Fluor 594-conjugated anti-mouse or rabbit IgG were used as secondary antibodies (Invitrogen). DNA was visualized by DAPI (4′,6-diamidino-2-phenylindole) staining. Immunostaining of the cell preparations was recorded by using an epifluorescence Zeiss Axioplan 2 microscope (Zeiss, Inc., Thornwood, NY) attached to a charge-coupled-device camera. In vitro kinase assay GST-tagged wild-type and geminin T25A mutant geminin were subcloned into pGEX, expressed in E. coli and purified. Aurora-A kinase was obtained from Millipore. Purified GST-tagged wild-type geminin or geminin T25A was incubated with Aurora-A in a kinase reaction buffer (25 mM Tris–HCl pH 7.5, 5 mM β-glycerophosphate, 2 mM DTT, 0.1 mM Na 3 VO 4 , 10 mM MgCl 2 and 0.1 mM ATP) supplemented with 5 μCi of [γ-32P] ATP at 30 °C for 60 min. The reactions were stopped with Laemmli buffer for 5 min at 95 °C. After the reaction mixtures were resolved by SDS–PAGE, the gels were stained with Coomassie brilliant blue, and were dried and subjected to autoradiography. BrdU staining Cells were treated with 33 μM BrdU for 30 min at 10.5 h after double thymidine block release ( Fig. 4a ). Cells were then fixed with 70% ethanol containing 10 mM glycine for 10 min, stained with mouse anti-BrdU primary antibody (Roche) and fluorescein-conjugated anti-mouse IgG secondary antibody (Roche), and analysed by indirect immunofluorescence. Nuclei were simultaneously counterstained with DAPI. The BrdU-positive nuclei were counted and plotted. Three independent counts ( n =150 cells each count) were used to calculate mean±s.d. How to cite this article: Tsunematsu, T. et al. Aurora-A controls pre-replicative complex assembly and DNA replication by stabilizing geminin in mitosis. Nat. Commun. 4:1885 doi: 10.1038/ncomms2859 (2013).